Bcl-wav and the mitochondrial calcium uniporter drive gastrula morphogenesis in zebrafish Bcl-2 proteins are acknowledged as key regulators of programmed cell death. However, increasing data suggest additional roles, including regulation of the cell cycle, metabolism and cytoskeletal dynamics. Here we report the discovery and characterization of a new Bcl-2-related multidomain apoptosis accelerator, Bcl-wav, found in fish and frogs. Genetic and molecular studies in zebrafish indicate that Bcl-wav and the recently identified mitochondrial calcium uniporter (MCU) contribute to the formation of the notochord axis by controlling blastomere convergence and extension movements during gastrulation. Furthermore, we found that Bcl-wav controls intracellular Ca 2+ trafficking by acting on the mitochondrial voltage-dependent anion channel, and possibly on MCU, with direct consequences on actin microfilament dynamics and blastomere migration guidance. Thus, from an evolutionary point of view, the original function of Bcl-2 proteins might have been to contribute in controlling the global positioning system of blastomeres during gastrulation, a critical step in metazoan development. Bcl-2 proteins are major regulators of programmed cell death. During early vertebrate development, they shape the embryo body through sustained cell homoeostasis and tissue morphogenesis. At the molecular level, Bcl-2 proteins act by controlling the mitochondrial release of cytotoxic molecules such as cytochrome- c , leading to caspase activation and subsequent apoptosis. The permeabilization of the outer mitochondrial membrane (OMM), which represents a key step during apoptosis, is regulated by the insertion of the apoptosis accelerators Bax and Bak and prevented by Bcl-2 and related apoptosis inhibitors [1] , [2] . In addition to apoptosis, mitochondria has a central role in intracellular calcium homoeostasis by rapidly transporting Ca 2+ from the cytosol to the mitochondrial matrix [3] , [4] . This process requires the passage of Ca 2+ ions through the voltage-dependent anion channel (VDAC) at the OMM [5] . At the inner mitochondrial membrane, this process is completed via the mitochondrial calcium uniporter (MCU), which was described only recently [6] , [7] . Members of the Bcl-2 family actively participate in the control of calcium homoeostasis by binding to VDAC and controlling its Ca 2+ permeability [8] . Despite these findings, the majority of studies have been performed in vitro , and the physiological relevance of this calcium control at the level of the whole organism, especially during the first steps of vertebrate development, remains unclear. Zebrafish has become a powerful model organism for studying the role of genes related to early vertebrate development and apoptosis [9] . During this stage, a set of morphogenetic movements known as convergence and extension (C&E) begins; these movements shape the embryo body in a co-ordinated fashion. C&E movements are characterized by blastomere migration from the ventral to the dorsal region and at the animal pole, resulting in the formation of the anteroposterior and mediolateral axes [10] . Interestingly, during these early stages, bcl-2 and related genes are actively transcribed, which suggests their implication in the zebrafish development [11] . Moreover, Ca 2+ signalling has a crucial role in early development, particularly during gastrulation [12] . Recently, we have characterized a Bcl-2-related anti-apoptotic protein, Nrz [13] . The Nrz protein controls the first morphogenetic movement, known as epiboly, during early zebrafish development [14] . At the molecular level, epiboly is achieved through Nrz-dependent intracellular calcium control, highlighting the emerging role of Bcl-2 proteins as multifunctional cell factors during early vertebrate development. Here we present the identification of the new apoptosis accelerator Bcl-wav, named for its expression in water-living vertebrates (anamniotes). The Bcl-wav protein shares structural and functional similarities, including its mitochondrial localization, with multidomain death accelerators. Knockdown of bclwav or mcu in zebrafish results in major alterations in the C&E movements of blastomeres during gastrulation, presumably due to alterations in F-actin dynamics. At later stages, we found that the maturation of the notochord and anteroposterior axis formation were compromised by bclwav or mcu silencing. At the molecular level, Bcl-wav interacted with both VDAC type 1 (VDAC1) and MCU, demonstrating that it is critical for mitochondrial Ca 2+ uptake. Finally, Bcl-wav and MCU controlled the overall blastomere positioning system during gastrulation via the regulation of intracellular calcium trafficking. Together, our data support the notion that the Bcl-2 proteins have key roles in early development by controlling actin microfilament dynamics and thus also cell movement. Expression of bclwav during zebrafish development We recently developed a set of structure-based hidden Markov model profiles specific for cellular and/or viral-encoded proteins that share the same three-dimensional fold as Bcl-2 [15] (ref.15). These novel models reliably identified Bcl-2 family-related proteins in a vast array of metazoans, including members with low sequence similarity. During the course of these studies, we discovered a previously uncharacterized open-reading frame present in the zebrafish genome, which we believed was likely to encode a new Bcl-2 homologue. Subsequent BLAST searches identified expressed sequence tags (ESTs) with significant similarity to the corresponding putative product in teleosts and anurans; however, no corresponding EST was found in birds or mammals. This sequence was thus named Bcl-wav, for ‘water-living anamniote vertebrates’ ( Fig. 1a ). The bclwav sequence can be found in GenBank under accession number GU350411.1 (NCBI NP_001165873). Local alignment matrices showed that the zebrafish and Xenopus Bcl-wav proteins clustered with multidomain Bcl-2 members, consistent with Bcl-wav primary sequence analyses, which identified four Bcl-2 homology (BH) domains and a C-terminal transmembrane (TM) domain ( Fig. 1b,c ). Moreover, secondary structure predictions revealed an all-alpha helical structure, which is typical of Bcl-2-like proteins ( Fig. 1c ). 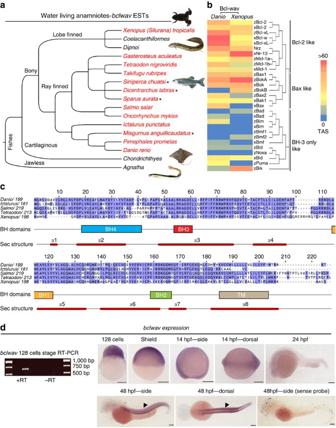Figure 1: Sequence and expression analysis of thebclwavgene. (a) Cladogram ofbclwav-orthologous ESTs retrieved from GenBank, indicating the restricted phylogenetic distribution of thebclwavgene in aquatic anamniotes. Partial (*) and totalbclwavESTs were found inDanio rerio,Pimephales promelas,Misgurnus anguillicaudatus,Oncorhynchus mykiss,Salmo salar,Gasterosteus aculeatus,Tetraodon nigroviridis,Takifugu rubripes,Dicentrarchus labrax,Siniperca chuatsi,Sparus aurata,Ictalurus punctatusandXenopus tropicalis(red lines). (b)In silicohybridization matrix representing the alignment ofD. rerio(Bcl-wav) andX. tropicalis(xBcl-wav)bclwavorthologs versus the Bcl-2-related proteins found in these two species. Coloured boxes indicate to the total alignment score (blue, no alignment; red, high alignment score (>60)). Bcl-wav and xBcl-wav cluster mainly with multidomain Bcl-2 members. (c) ClustalW alignment of Bcl-wav primary structures in multiple species. Identical and similar residues are boxed in blue and cyan, respectively. The positions of conserved BH1-BH4 domains and of the C-terminal TM domain are indicated by coloured boxes below the sequences, and the locations of the predicted alpha helices are indicated by red stripes. (d) Reverse transcriptase PCR of polyA+ RNA extracted from whole embryos before the mid-blastula transition (MBT).Bclwavexpression was detected in embryos before the MBT (+RT) (top left panel). A reaction lacking the RT enzyme (−RT) was used as a negative control. Top right and bottom panels showbclwavwhole-mountin situhybridization. Before MBT (128 cells), at the shield (6 hpf) and 14 hpf stages,bclwavis ubiquitously expressed. At 24 hpf,bclwavexpression decreases. In addition, at 48 hpf,bclwavis highly expressed in the somites (black arrowheads). A negative control at 48 hpf using a sense probe is shown in the bottom right-outermost panel. Scale bar, 200 μm. Figure 1: Sequence and expression analysis of the bclwav gene. ( a ) Cladogram of bclwav -orthologous ESTs retrieved from GenBank, indicating the restricted phylogenetic distribution of the bclwav gene in aquatic anamniotes. Partial (*) and total bclwav ESTs were found in Danio rerio , Pimephales promelas , Misgurnus anguillicaudatus , Oncorhynchus mykiss , Salmo salar , Gasterosteus aculeatus , Tetraodon nigroviridis , Takifugu rubripes , Dicentrarchus labrax , Siniperca chuatsi , Sparus aurata , Ictalurus punctatus and Xenopus tropicalis (red lines). ( b ) In silico hybridization matrix representing the alignment of D. rerio (Bcl-wav) and X. tropicalis (xBcl-wav) bclwav orthologs versus the Bcl-2-related proteins found in these two species. Coloured boxes indicate to the total alignment score (blue, no alignment; red, high alignment score (>60)). Bcl-wav and xBcl-wav cluster mainly with multidomain Bcl-2 members. ( c ) ClustalW alignment of Bcl-wav primary structures in multiple species. Identical and similar residues are boxed in blue and cyan, respectively. The positions of conserved BH1-BH4 domains and of the C-terminal TM domain are indicated by coloured boxes below the sequences, and the locations of the predicted alpha helices are indicated by red stripes. ( d ) Reverse transcriptase PCR of polyA+ RNA extracted from whole embryos before the mid-blastula transition (MBT). Bclwav expression was detected in embryos before the MBT (+RT) (top left panel). A reaction lacking the RT enzyme (−RT) was used as a negative control. Top right and bottom panels show bclwav whole-mount in situ hybridization. Before MBT (128 cells), at the shield (6 hpf) and 14 hpf stages, bclwav is ubiquitously expressed. At 24 hpf, bclwav expression decreases. In addition, at 48 hpf, bclwav is highly expressed in the somites (black arrowheads). A negative control at 48 hpf using a sense probe is shown in the bottom right-outermost panel. Scale bar, 200 μm. Full size image To investigate bclwav expression, we performed reverse transcriptase PCR experiments on zebrafish embryos. Bclwav mRNA could be detected as early as the 128-cell stage, that is, before the mid-blastula transition [16] , indicating that the bclwav transcript is maternally inherited ( Fig. 1d ). Bclwav expression was further analysed by in situ hybridization using two non-overlapping bclwav probes and one full-length bclwav probe. The same expression pattern was obtained with all three probes ( Fig. 1d ). Indeed, bclwav was ubiquitously expressed up to 14 h post fertilization (hpf), whereas at later stages (36–48 hpf) its expression became somite-specific. Interestingly, these results corroborated the fact that bclwav ESTs were found in muscle tissue ( Salmo salar , smus1-014AD07.g1 and Xenopus tropicalis , XP_002940781.1), suggesting a conserved expression pattern across species. Bcl-wav is a mitochondrial pro-apoptotic Bcl-2 family member To gain insight into the function of Bcl-wav, we first investigated its subcellular distribution in vitro . Confocal microscopy analyses showed that Bcl-wav was mainly localized in the mitochondria (85±6.8% co-localization with Mitotracker, n =5; measured using Zeiss LSM 780 Zen software); however, the Bcl-wavΔTM mutant, which lacked the C-terminal TM domain, was cytosolic ( Fig. 2a,b and Supplementary Fig. S1a,b ). Analyses of purified mitochondria from zebrafish embryos injected with in vitro -synthesized mRNAs encoding either full-length Bcl-wav or the Bcl-wavΔTM deletion mutant showed that Bcl-wavΔTM was unable to localize in the mitochondrial fraction ( Supplementary Fig. S1b ). Notably, deleting the BH4 domain did not affect Bcl-wav subcellular localization ( Fig. 2b ). Furthermore, the Bcl-wav protein appeared to be tightly anchored to the mitochondria, as demonstrated by an Na 2 CO 3 treatment assay ( Fig. 2c ). 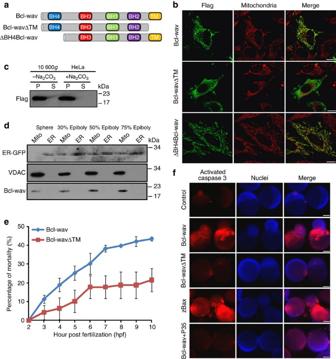Figure 2: Bcl-wav is a mitochondrial pro-apoptotic protein. (a) Schematic drawing of recombinant proteins: full-length Bcl-wav, Bcl-wavΔTM and ΔBH4Bcl-wav. The BH and TM domains are shown as coloured boxes. (b) Analysis of Bcl-wav subcellular localization by confocal microscopy in HeLa cells transiently transfected with pCS2+Flag-Bcl-wav, pCS2+Flag-Bcl-wavΔTM and pCS2+Flag-ΔBH4Bcl-wav expressing Flag-Bcl-wav, Flag-Bcl-wavΔTM and Flag-ΔBH4Bcl-wav fusion proteins, respectively. Mitochondria were labelled using Mitotracker red dye, and Flag fusion proteins were detected using an anti-Flag antibody. In contrast to Flag-Bcl-wavΔTM, which is localized in the cytosol, Flag-Bcl-wav and Flag-ΔBH4Bcl-wav co-localize with mitochondria. Scale bar, 5 μm. (c) Flag-Bcl-wav is inserted into the mitochondrial membrane. Purified mitochondria from Flag-Bcl-wav-expressing cells were treated with sodium carbonate and immunoblotted with the anti-Flag antibody. Flag-Bcl-wav was found in the mitochondrial pellet (P) containing membrane-inserted proteins and was not found in the supernatant (S). (d) Bcl-wav is a mitochondrial zebrafish protein. Subcellular fractionation of YSL mitochondria and YSL endoplasmic reticulum (ER) of embryos expressing ER-GFP at the sphere stage and at 30%, 50% and 75% epiboly. Bcl-wav was detected in the mitochondrial fraction (Mito) and accumulates during gastrulation. VDAC and GFP antibodies were used as mitochondrial and ER markers, respectively. (e) The effect ofbclwavoverexpression on the mortality of zebrafish embryos. In contrast tobclwavΔTMmRNA,bclwavmRNA injection (100 ng/μl) into 1–4 cell stage embryos induces early mortality during gastrulation (mean±s.d.; three independent experiments). (f)Bclwavoverexpression promotes caspase 3 activation in zebrafish embryos at 50% epiboly. Left panels: activated caspase 3 staining in embryos injected at the one-cell stage withegfp(control),zbax,bcl-wavΔtm,bclwavandbclwavplusp35mRNAs. Embryos were observed at 30–50% epiboly. Middle panels: the same embryos were stained with Hoechst reagent to visualize the nuclei. Right panels: merged images of stained embryos.Bclwavoverexpression induces YSL-specific caspase 3 activation (48%), which is abrogated by p35 co-injection (8%). Scale bar, 200 μm. Full scans of western blots can be found inSupplementary Fig. S9. Figure 2: Bcl-wav is a mitochondrial pro-apoptotic protein. ( a ) Schematic drawing of recombinant proteins: full-length Bcl-wav, Bcl-wavΔTM and ΔBH4Bcl-wav. The BH and TM domains are shown as coloured boxes. ( b ) Analysis of Bcl-wav subcellular localization by confocal microscopy in HeLa cells transiently transfected with pCS2+Flag-Bcl-wav, pCS2+Flag-Bcl-wavΔTM and pCS2+Flag-ΔBH4Bcl-wav expressing Flag-Bcl-wav, Flag-Bcl-wavΔTM and Flag-ΔBH4Bcl-wav fusion proteins, respectively. Mitochondria were labelled using Mitotracker red dye, and Flag fusion proteins were detected using an anti-Flag antibody. In contrast to Flag-Bcl-wavΔTM, which is localized in the cytosol, Flag-Bcl-wav and Flag-ΔBH4Bcl-wav co-localize with mitochondria. Scale bar, 5 μm. ( c ) Flag-Bcl-wav is inserted into the mitochondrial membrane. Purified mitochondria from Flag-Bcl-wav-expressing cells were treated with sodium carbonate and immunoblotted with the anti-Flag antibody. Flag-Bcl-wav was found in the mitochondrial pellet (P) containing membrane-inserted proteins and was not found in the supernatant (S). ( d ) Bcl-wav is a mitochondrial zebrafish protein. Subcellular fractionation of YSL mitochondria and YSL endoplasmic reticulum (ER) of embryos expressing ER-GFP at the sphere stage and at 30%, 50% and 75% epiboly. Bcl-wav was detected in the mitochondrial fraction (Mito) and accumulates during gastrulation. VDAC and GFP antibodies were used as mitochondrial and ER markers, respectively. ( e ) The effect of bclwav overexpression on the mortality of zebrafish embryos. In contrast to bclwavΔTM mRNA, bclwav mRNA injection (100 ng/μl) into 1–4 cell stage embryos induces early mortality during gastrulation (mean±s.d. ; three independent experiments). ( f ) Bclwav overexpression promotes caspase 3 activation in zebrafish embryos at 50% epiboly. Left panels: activated caspase 3 staining in embryos injected at the one-cell stage with egfp (control), zbax , bcl-wavΔtm , bclwav and bclwav plus p35 mRNAs. Embryos were observed at 30–50% epiboly. Middle panels: the same embryos were stained with Hoechst reagent to visualize the nuclei. Right panels: merged images of stained embryos. Bclwav overexpression induces YSL-specific caspase 3 activation (48%), which is abrogated by p35 co-injection (8%). Scale bar, 200 μm. Full scans of western blots can be found in Supplementary Fig. S9 . Full size image Next, we directly evaluated the subcellular localization of the endogenous Bcl-wav protein in zebrafish embryos using a rabbit polyclonal antibody. To this end, mitochondria and endoplasmic reticulum (ER) fractions purified from the yolk syncytial layer (YSL) of embryos at various stages of epiboly were analysed; these experiments showed that Bcl-wav was already present at the sphere stage and gradually accumulated during gastrulation ( Fig. 2c,d ). Together, these findings showed that Bcl-wav is a resident mitochondrial protein that is presumably inserted into the OMM via its hydrophobic TM domain. The activity of Bcl-wav was then analysed further. The ectopic expression of Bcl-wav in zebrafish embryos and HeLa cells demonstrated its capacity to activate caspase 3, in contrast to the Bcl-wavΔTM mutant, which failed to do so ( Fig. 2e,f and Supplementary Fig. S2a–c ). Moreover, caspase activation was prevented by the apoptosis inhibitors zBcl-xL and Nrz ( Supplementary Fig. S2b ). Notably, the ΔBH4 deletion mutant was still found to activate caspase 3 and lead to an increase in cleaved poly(ADP) ribose polymerase (PARP), a target of caspases during apoptosis, indicating that the BH4 domain is dispensable for apoptosis induction by Bcl-wav ( Supplementary Fig. S2c ). In addition, Bcl-wav appeared to activate caspase 3 in a Bax/Bak-dependent manner, as shown using bax/bak -deficient mouse embryo fibroblasts ( Supplementary Fig. S2d ). Interestingly, the Bcl-wav/Bax interaction was detected by co-immunoprecipitation assays in HeLa cells ( Supplementary Fig. S2e ). These results were confirmed by experiments in a yeast model, which showed that Bcl-wav could activate Bax and promote cytochrome- c release ( Supplementary Fig. S3 ). Overall, these data suggest that Bcl-wav is a new potential death accelerator that shares structural similarities with multidomain Bcl-2 family members. Bclwav knockdown leads to major developmental defects Knockdown experiments with morpholinos were carried out to further investigate Bcl-wav role during development. In these experiments, anti- bclwav morpholinos were co-injected together with an anti- p53 morpholino ( p53 -MO) to abolish the non-specific induction of p53-dependent cell death, a frequent off-target effect of morpholinos [17] . Notably, two different morpholinos targeting distinct regions of the bclwav gene were used ( bclwav MO1 and bclwav MO2), whereas a control morpholino (5mis-MO, termed controlMO) was used as a negative control. The efficiency of the bclwav MOs was confirmed by immunoblotting of mitochondrial extracts of zebrafish embryos at 50% epiboly ( Fig. 3a ). Bclwav knockdown induced major developmental abnormalities, and similar phenotypes were obtained with both morpholinos ( Fig. 3b ). Most bclwav morphants (86%, n =579) ( Fig. 3c and Supplementary Fig. S4a ) were able to complete somitogenesis but showed anteroposterior axis reduction and abnormal somites. Moreover, the use of SonicHedgehogGFP ( shh:gfp ) transgenic embryos showed that bclwav morphants exhibited misplaced and bent notochords, randomly shifted to either the right or the left, giving rise to a typical bending of the embryo at 24 hpf ( Fig. 3d–f ). These results were confirmed by in situ hybridization in 14 hpf embryos using col2.1 as a probe, highlighting the curvature of the notochord ( Fig. 3e ). Contrary to bclwav morphants, most controls appeared to be normal (94%, n =141) ( Fig. 3c ). A minority of bclwav morphants (9%) exhibited an even more severe phenotype, as illustrated by premature developmental arrest shortly after the beginning of somitogenesis. The specificity of the bclwav morphant phenotype was confirmed by co-injecting bclwav mRNA with bclwav MO. Under these conditions, the injected embryo phenotype (86% normal, n =123) was similar to that of the controls ( Fig. 3c ). In such complementation experiments, mRNA of the caspase inhibitor p35 was co-injected with bclwav mRNA to prevent apoptosis due to Bcl-wav protein accumulation. Interestingly, at later stages (26 hpf), the somite alterations observed in bclwav morphants were correlated with a marked increase in caspase-dependent cell death events, as well as severe disorganization of the actin fibres in the somites, compared with control embryos ( Supplementary Fig. S4b,c ). 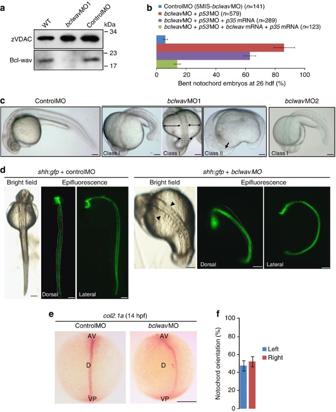Figure 3:Bclwavknockdown leads to major developmental defects. (a) Immunoblot analysis ofbclwavmorpholino efficiency in mitochondria purified from WT embryos and embryos injected withbclwavMO1 and controlMO at 50% epiboly (5 hpf) using anti-Bcl-wav polyclonal antibody. A specific signal that disappears following the injection ofbclwavMO was detected. VDAC was used as an internal loading control. (b) Histograms representing the percentage of bent notochord phenotypes at 26 hpf in controlMO (5Mis-MO+p53-MO) embryos versusbclwavmorphants injected withbclwavorp35mRNAs. The ectopic expression of p35 does not prevent thebclwavMO effect, indicating a caspase-independent phenomenon. Co-injection ofbclwavmRNA (as well asp35mRNA) together withbclwavMO restores normal development (mean±s.d.; three independent experiments). (c)Bclwavknockdown phenotype at 26 hpf. Embryos injected with negative controlMO were normal (left panel). In contrast, embryos injected with antisense morpholinos (bclwavMO1+p53-MO orbclwavMO2+p53-MO) show similar class I (77%) and class II (9%) abnormal phenotypes. Embryos with the class I phenotype (left and middle panels) exhibit abnormal somites (black arrowheads), as well as bent notochord and anteroposterior axis (two-ended arrows). The class II phenotype is characterized by a major developmental delay, showing the lack of anteroposterior differentiation at 26 hpf (right panel, black arrow). Scale bar, 200 μm. (d) Visualization of the bent notochord phenotype in thebclwavknockdown mutant usingshh:gfpembryos compared with controlMO. Inbclwavmorphants, the notochord is shifted laterally (right panel), near the ear. Scale bar, 200 μm. (e)Col2.1awhole-mountin situhybridization at 14 hpf. In contrast to controlMO embryos,bclwavMO embryos exhibit a deviation of thecol2.1asignal relative to the anteroposterior axis. AP, animal pole; D, dorsal; VP, vegetal pole. Scale bar, 200 μm. (f) Histogram representing the percentage of individuals with notochord deviation (to the right or to the left) inbclwavMO embryos at 26 hpf (mean±s.d.; three independent experiments). Full scans of the western blots are provided inSupplementary Fig. S9. Figure 3: Bclwav knockdown leads to major developmental defects. ( a ) Immunoblot analysis of bclwav morpholino efficiency in mitochondria purified from WT embryos and embryos injected with bcl wavMO1 and controlMO at 50% epiboly (5 hpf) using anti-Bcl-wav polyclonal antibody. A specific signal that disappears following the injection of bclwav MO was detected. VDAC was used as an internal loading control. ( b ) Histograms representing the percentage of bent notochord phenotypes at 26 hpf in controlMO (5Mis-MO +p53 -MO) embryos versus bclwav morphants injected with bclwav or p35 mRNAs. The ectopic expression of p35 does not prevent the bclwav MO effect, indicating a caspase-independent phenomenon. Co-injection of bclwav mRNA (as well as p35 mRNA) together with bclwav MO restores normal development (mean±s.d. ; three independent experiments). ( c ) Bclwav knockdown phenotype at 26 hpf. Embryos injected with negative controlMO were normal (left panel). In contrast, embryos injected with antisense morpholinos ( bclwav MO1+ p53- MO or bclwav MO2+ p53- MO) show similar class I (77%) and class II (9%) abnormal phenotypes. Embryos with the class I phenotype (left and middle panels) exhibit abnormal somites (black arrowheads), as well as bent notochord and anteroposterior axis (two-ended arrows). The class II phenotype is characterized by a major developmental delay, showing the lack of anteroposterior differentiation at 26 hpf (right panel, black arrow). Scale bar, 200 μm. ( d ) Visualization of the bent notochord phenotype in the bclwav knockdown mutant using shh:gfp embryos compared with controlMO. In bclwav morphants, the notochord is shifted laterally (right panel), near the ear. Scale bar, 200 μm. ( e ) Col2.1a whole-mount in situ hybridization at 14 hpf. In contrast to controlMO embryos, bclwav MO embryos exhibit a deviation of the col2.1a signal relative to the anteroposterior axis. AP, animal pole; D, dorsal; VP, vegetal pole. Scale bar, 200 μm. ( f ) Histogram representing the percentage of individuals with notochord deviation (to the right or to the left) in bclwav MO embryos at 26 hpf (mean±s.d. ; three independent experiments). Full scans of the western blots are provided in Supplementary Fig. S9 . Full size image Overall, the results of these experiments suggest that bclwav knockdown causes developmental retardation and notochord bending, as well as somite malformation. Interestingly, ectopic expression of p35 failed to restore normal development (bent notochord embryos: 63%, n =289) ( Fig. 3c ). These observations suggest that the bclwav MO phenotype did not result from caspase activation. Bcl-wav controls C&E cell movements during gastrulation In vertebrates, the co-ordinated movements of the blastomeres during C&E ensure the establishment of the anteroposterior axis and the embryo body plan. We hypothesized that the malformations observed at later stages in bclwav morphants might result from impaired gastrulation. We first analysed the anterior progression of the dorsal progenitor cells during gastrulation. Bclwav silencing resulted in a significant shortening of the embryos, suggesting a defect in morphogenetic movements during gastrulation ( Fig. 4a,b ). We next analysed the progression of mesoderm progenitors, which contributes to the formation of the notochord, by performing in situ hybridization at 75% epiboly and using no tail ( ntl ) as a marker. In bclwav morphants, ntl -positive cells showed a disturbed anteroposterior distribution in the dorsal region ( Fig. 4c ). The length (l/L) and width (w/W) ratios of bclwav morphants (l/L=0.45±0.04 and w/W=0.32±0.02) were significantly lower and higher, respectively, than those of the controls (l/L=0.61±0.03 and w/W=0.25±0.02), suggesting a defect in the migration of these cells during gastrulation ( Fig. 4d ). Using time-lapse videomicroscopy, we specifically tracked the progression of the paraxial mesoderm, which undergoes C&E movements. The net progression of mesoderm cells towards the dorsal meridian axis was significantly affected in bclwav morphants ( Fig. 4e ). Analyses of their migration paths showed that, in contrast to the synchronously migrating control cells, the migration paths of many mesoderm cells in bclwav morphants were random ( Fig. 4f ). These results showed that although the mesoderm precursor cells migrated at a normal velocity in bclwav morphants, their progression towards the dorsal meridian axis was compromised. Because such alterations could be the consequence of cell autonomous or non-cell-autonomous phenomena, we set up a series of transplant experiments to observe the behaviour of morphant blastomeres in a wild-type (WT) environment. When implanted into WT receiving embryos, blastomeres from control donors were found to spread along the dorsal axis due to cellular intercalation ( Fig. 4g ). In contrast, transplanted blastomeres from morphant embryos were unable to undergo such spreading, which resulted in altered C&E movements in the dorsal region of the morphant embryos ( Fig. 4h ). These results suggest that the origins of the observed defects were, at least in part, cell autonomous. 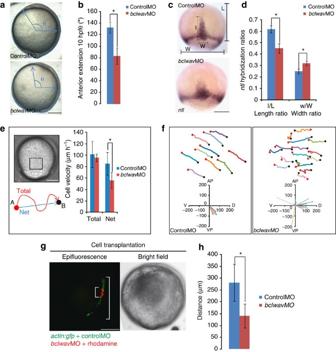Figure 4: Effect ofbclwavknockdown on cell movement during C&E movements. (a) Representative bright field images of controlMO andbclwavMO at the tail bud stage, showing the delay in the progression of dorsal progenitors as measured by the angle between the head and the equator (θ). Scale bar, 200 μm. (b) Histograms quantifying theθangle difference between control embryos andbclwavmorphants.Bclwavsilencing induces a significant reduction in anterior extension (mean±s.d.; three independent experiments; *P<0.01, Student’st-test). (c)Ntlwhole-mountin situhybridization at 75% epiboly. Thentl-positive mesoderm cells inbclwavmorphants show disturbed anteroposterior migration at the dorsal pole relative to controlMO embryos.Ntl-positive signal length (l/L) and width (w/W) ratios are used to calculate mesoderm progression. Scale bar, 200 μm. (d) Histograms representing the l/L and w/W ratios of controlMO embryos andbclwavmorphants at the 75% epiboly stage (mean±s.d.; three independent experiments; *P<0.01, Student’st-test). (e) Histograms representing the quantification of the total velocity (total distance, μm h−1) and net velocity (net dorsal progression, μm h−1) of the lateral mesodermal cells during C&E movements (at 75% epiboly). The net velocity of the mesodermal cells is significantly lower inbclwavMO than in control embryos (mean±s.d.; three independent experiments; *P<0.01, Student’st-test). Scale bar, 200 μm. (f) Cell paths and vector projections of isolated mesodermal cells observed during C&E movements at the 75% epiboly stage in embryos injected with controlMO orbclwavMO. Compared with the control cells, which migrate synchronously,bclwavMO lateral mesodermal cells exhibit more random migration paths. Images and diagrams are oriented as follows: AP, animal pole; D, dorsal; V, ventral; and VP, vegetal pole. (g) Observation of GFP-expressing cells injected with controlMO and morphant (bclwavMO+rhodamine) cells transplanted into WT embryos. Control cells (green) show a greater distribution along the dorsal axis than thebclwav-silenced cells (red). Scale bar, 200 μm. (h) Histograms showing the distance covered by controlMO cells versusbclwav-silenced cells (controlMO:n=13 embryos andbclwavMO:n=10 embryos) (mean±s.d.; *P<0.01, Student’st-test). Figure 4: Effect of bclwav knockdown on cell movement during C&E movements. ( a ) Representative bright field images of controlMO and bclwav MO at the tail bud stage, showing the delay in the progression of dorsal progenitors as measured by the angle between the head and the equator ( θ ). Scale bar, 200 μm. ( b ) Histograms quantifying the θ angle difference between control embryos and bclwav morphants. Bclwav silencing induces a significant reduction in anterior extension (mean±s.d. ; three independent experiments; * P <0.01, Student’s t -test). ( c ) Ntl whole-mount in situ hybridization at 75% epiboly. The ntl -positive mesoderm cells in bclwav morphants show disturbed anteroposterior migration at the dorsal pole relative to controlMO embryos. Ntl -positive signal length (l/L) and width (w/W) ratios are used to calculate mesoderm progression. Scale bar, 200 μm. ( d ) Histograms representing the l/L and w/W ratios of controlMO embryos and bclwav morphants at the 75% epiboly stage (mean±s.d. ; three independent experiments; * P <0.01, Student’s t -test). ( e ) Histograms representing the quantification of the total velocity (total distance, μm h −1 ) and net velocity (net dorsal progression, μm h −1 ) of the lateral mesodermal cells during C&E movements (at 75% epiboly). The net velocity of the mesodermal cells is significantly lower in bclwav MO than in control embryos (mean±s.d. ; three independent experiments; * P <0.01, Student’s t -test). Scale bar, 200 μm. ( f ) Cell paths and vector projections of isolated mesodermal cells observed during C&E movements at the 75% epiboly stage in embryos injected with controlMO or bclwav MO. Compared with the control cells, which migrate synchronously, bclwav MO lateral mesodermal cells exhibit more random migration paths. Images and diagrams are oriented as follows: AP, animal pole; D, dorsal; V, ventral; and VP, vegetal pole. ( g ) Observation of GFP-expressing cells injected with controlMO and morphant ( bclwav MO+rhodamine) cells transplanted into WT embryos. Control cells (green) show a greater distribution along the dorsal axis than the bclwav -silenced cells (red). Scale bar, 200 μm. ( h ) Histograms showing the distance covered by controlMO cells versus bclwav -silenced cells (controlMO: n =13 embryos and bclwav MO: n =10 embryos) (mean±s.d. ; * P <0.01, Student’s t -test). Full size image Bclwav knockdown alters F-actin dynamics during gastrulation Cell migration depends strongly on actin microfilament dynamics. We thus monitored actin polymerization in control embryos and bclwav morphants using a green fluorescent protein (GFP)-tagged peptide that is able to bind F-actin (lifeactGFP). In control embryos, lateral mesodermal cells exhibited F-actin protrusions at the leading edge, which were oriented in the posterior–dorsal direction ( Fig. 5a–d and Supplementary Movie 1 ). In contrast, F-actin protrusions in bclwav morphants were more randomly oriented ( Fig. 5a–d and Supplementary Movie 2 ). Moreover, F-actin dynamics were also affected by bclwav silencing. In control embryos, F-actin protrusions were highly dynamic by polymerizing and depolymerizing periodically (average period: 80 s), whereas these protrusions persisted for much longer periods in bclwav morphants, indicating that the dynamics of the protrusions were severely altered ( Fig. 5a,b ). Overall, these results suggest that bclwav silencing led to mesoderm C&E migration defects as a consequence of impaired actin microfilament dynamics and polarity. 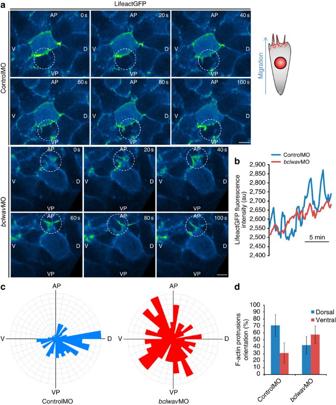Figure 5:Bclwavknockdown disrupts actin protrusion dynamics and orientation. (a) Confocal spinning disk microscopy analysis of F-actin dynamics in controlMO andbclwavmorphants expressinglifeactgfpat the 75% epiboly stage. F-actin-enriched cell protrusions are essential for cell migration. Cells frombclwavMO-injected embryos show altered F-actin polymerization positioning and dynamics (white circles). Image acquisition was performed on a single confocal section to visualize polymerized actin in lateral mesodermal cells. Scale bar, 10 μm. (b) Graph representing the fluorescence intensity of LifeactGFP-positive cells over 20 min of tracking. Control cells show periodic increases and decreases in fluorescence intensity corresponding to F-actin polymerization and depolymerization. Inbclwav-silenced cells, these F-actin dynamics are strongly altered. (c) Circular rose diagrams of controlMO versusbclwavMO embryos representing the orientation of actin protrusions. These diagrams show the frequency of protrusions in a given orientation. The directionality of the F-actin protrusions is more random inbclwavMO embryos than in controlMO embryos. Diagrams are oriented as follows: AP, animal pole; D, dorsal; V, ventral; VP, vegetal pole. (d) Histograms representing F-actin protrusion orientations. The F-actin protrusions of control embryos are mainly oriented in the dorsal quadrant, whereas those inbclwavmorphants are inverted (that is, in the ventral quadrant) (mean±s.d.;n=111 and 141 cells for controlMO andbclwavMO, respectively; three independent experiments). Figure 5: Bclwav knockdown disrupts actin protrusion dynamics and orientation. ( a ) Confocal spinning disk microscopy analysis of F-actin dynamics in controlMO and bclwav morphants expressing lifeactgfp at the 75% epiboly stage. F-actin-enriched cell protrusions are essential for cell migration. Cells from bclwav MO-injected embryos show altered F-actin polymerization positioning and dynamics (white circles). Image acquisition was performed on a single confocal section to visualize polymerized actin in lateral mesodermal cells. Scale bar, 10 μm. ( b ) Graph representing the fluorescence intensity of LifeactGFP-positive cells over 20 min of tracking. Control cells show periodic increases and decreases in fluorescence intensity corresponding to F-actin polymerization and depolymerization. In bclwav -silenced cells, these F-actin dynamics are strongly altered. ( c ) Circular rose diagrams of controlMO versus bclwav MO embryos representing the orientation of actin protrusions. These diagrams show the frequency of protrusions in a given orientation. The directionality of the F-actin protrusions is more random in bclwav MO embryos than in controlMO embryos. Diagrams are oriented as follows: AP, animal pole; D, dorsal; V, ventral; VP, vegetal pole. ( d ) Histograms representing F-actin protrusion orientations. The F-actin protrusions of control embryos are mainly oriented in the dorsal quadrant, whereas those in bclwav morphants are inverted (that is, in the ventral quadrant) (mean±s.d. ; n =111 and 141 cells for controlMO and bclwav MO, respectively; three independent experiments). Full size image Bcl-wav sustains mitochondrial Ca 2+ uptake via VDAC1 During gastrulation, Bcl-wav protein is exclusively mitochondrial. This led us to hypothesize that the observed C&E defects could be due to mitochondrial dysfunction. Surprisingly, none of the mitochondrial parameters analysed, including mitochondrial transmembrane potential (ΔΨm), ROS production, mitochondrial respiration or cytochrome- c release, appeared to be affected in bclwav morphants ( Supplementary Fig. S5 ). However, when mitochondrial Ca 2+ levels were measured using a dedicated fluorescent dye (Rhod-FF), we detected a significant decrease in mitochondrial Ca 2+ content compared with control embryos ( Fig. 6a–c ). Moreover, this mitochondrial Ca 2+ decrease was correlated with an increase in cytosolic [Ca 2+ ] and a decrease in the mitochondria to cytosolic calcium ratio, suggesting that Bcl-wav might control Ca 2+ fluxes between mitochondria and the cytosol ( Fig. 6a–c and Supplementary Movies 3 and 4 ). To test this hypothesis further, we evaluated the effect of ectopic Bcl-wav expression on mitochondrial Ca 2+ uptake following an artificial increase in cytosolic Ca 2+ levels in HeLa cells. Bcl-wav expression significantly increased mitochondrial Ca 2+ uptake ( Fig. 6d,e ). We next evaluated the effect of bclwav knockdown on the capacity of purified mitochondria from zebrafish embryos to take up exogenous Ca 2+ (20 μM). Bclwav -deficient mitochondria had a decreased Ca 2+ uptake capacity compared with control mitochondria ( Fig. 6f,g ). VDAC1 is a major component of the apoptosis machinery; the pharmacological inhibition of VDAC using 2 mM NADH completely abolished Ca 2+ entry into mitochondria, illustrating the critical role of VDAC as a Ca 2+ channel [5] , [18] , [19] ( Fig. 6f,g ). It was previously shown that Bcl-2 proteins, including Bcl-xL, could interact with VDAC [20] and modulate its activity via the BH4 domain [21] . We thus evaluated whether Bcl-wav can interact with VDAC1. To this end, Flag-tagged Bcl-wav was ectopically expressed in zebrafish embryos. Immunoprecipitation assays performed using purified mitochondria from embryos overexpressing Flag-Bcl-wav showed that full-length Bcl-wav interacted with endogenous zVDAC1 ( Fig. 6h ). Interestingly, Bcl-wav was also found to interact with endogenous VDAC1 in HeLa cells ( Fig. 6i ), which might be expected because zebrafish and human VDAC1 are highly conserved (amino acid sequence identity: 85.5%). To determine whether Bcl-wav interacted with VDAC1 via its BH4 domain, immunoprecipitation assays in HeLa cells were also performed with Bcl-wav-deletion mutants in addition to full-length Bcl-wav. As shown in Fig. 6i , full-length Bcl-wav and Bcl-wavΔTM interacted with VDAC1. Although no interaction with ΔBH4Bcl-wav was detected, the BH4 domain alone interacted with VDAC1. In addition, in bclwav morphants, the ΔBH4Bcl-wav-deletion mutant neither restored normal development ( Fig. 6j ) nor prevented increases in cytosolic Ca 2+ ( Fig. 6k ), in contrast to full-length Bcl-wav. This result suggests that the Bcl-wav/zVDAC1 interaction was functionally significant. Together, these findings suggest that Bcl-wav may control mitochondrial Ca 2+ uptake via zVDAC1 during zebrafish gastrulation. Most interestingly, zBcl-xL completely reversed the effect of Bcl-wav on mitochondrial Ca 2+ uptake ( Fig. 6c,d ). Indeed, the ability of zBcl-xL to counteract the effect of Bcl-wav on Ca 2+ uptake might also depend on VDAC1, given that Bcl-xL has previously been shown to bind to VDAC [21] , [22] , [23] . 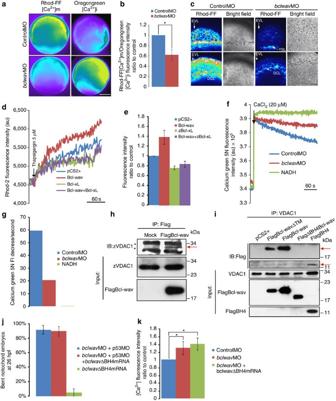Figure 6: Bcl-wav binds to zVDAC1viaits BH4 domain and controls mitochondrial calcium uptake. (a) Epifluorescence microscopy images of embryos at 75% epiboly stained with Rhod-FF or Oregon Green Bapta-1 AM fluorescent dyes measuring mitochondrial and cytosolic [Ca2+], respectively. False colour was applied to visualize the differences in the fluorescence intensities reflecting [Ca2+] changes. Dark blue: low [Ca2+]; yellow: high [Ca2+]. Scale bar, 200 μm. (b) Histograms showing fold changes in the Rhod-FF/Oregon Green Bapta-1 AM fluorescence intensities ofbclwavmorphants compared with controlMO (mean±s.d.; three independent experiments; *P<0.01, Student’st-test). (c) Confocal stacks of controlMO versusbclwavMO embryos stained with Rhod-FF dye at 75% epiboly. The enveloping cell layer (EVL), deep cell layer (DCL) and YSL of the embryo were analysed. Fluorescence intensities were visualized with false colour. Scale bar, 50 μm. (d) Representative response of transfected HeLa cells loaded with the mitochondrial Ca2+-sensitive dye Rhod-2. Mitochondrial Ca2+uptake was stimulated with 5 μM thapsigargin (black arrow). Scale bar, 60 s. (e) Histograms depicting the quantitative response of the cells to 5 μM thapsigargin (mean±s.d.; three independent experiments). (f) Analysis of the capacity of purified mitochondria frombclwavMO-, controlMO- or NADH (2 mM)-treated embryos (75% epiboly) to take up exogenous Ca2+(20 μM CaCl2). Calcium Green 5N fluorescent dye was used to measure the decrease in extramitochondrial [Ca2+], which directly reflects the mitochondrial uptake. Results are representative of two independent experiments. Scale bar, 60 s. (g) Histogram showing the capacity of purified mitochondria to uptake exogenous Ca2+as represented by a decrease in Oregon Green 5N fluorescence intensity (FI)/second. Results are representative of two independent experiments. (h) Bcl-wav co-immunoprecipitates with endogenous zVDAC1 in purified mitochondria from zebrafish embryos. Immunoprecipitations were performed using homogeneity-purified mitochondrial extracts from embryos (30% epiboly). Left lane (Mock), non-injected embryos; right lane (Flag-Bcl-wav), embryos injected with Flag-taggedbclwavtranscripts. In both samples, two non-specific bands are revealed by the anti-VDAC1 antibody, the lower corresponding to the immunoglobulin light chain (black stars); however, in the sample prepared from embryos injected with Flag-taggedbclwavtranscripts, a 34-kDa band corresponding to zVDAC1 can be detected (red arrow). (i) Bcl-wav interacts with endogenous VDAC1 via its BH4 domainin cellulo. Immunoprecipitation experiments were performed with protein extracts from transfected HeLa cells. Flag-Bcl-wav and Flag-Bcl-wavΔTM were both able to interact with VDAC1 (upper red arrow) but not Flag-ΔBH4Bcl-wav; the FlagBH4 peptide domain also interacted with VDAC1 (lower red arrow). (j) Histograms showing the percentage of embryos with the bent notochord phenotype (26 hpf) amongbclwavmorphants co-injected withΔBH4bclwavmRNA orΔBH4bclwavmRNA alone (mean±s.d.; three independent experiments). (k) Histograms indicating the fold changes in Oregon Green Bapta-1 fluorescence intensity ofbclwavmorphants injected or not withΔBH4BclwavmRNA compared with controlMO (mean±s.d.; three independent experiments; *P<0.01, Student’st-test). Full scans of western blots can be found inSupplementary Fig. S10. Figure 6: Bcl-wav binds to zVDAC1 via its BH4 domain and controls mitochondrial calcium uptake. ( a ) Epifluorescence microscopy images of embryos at 75% epiboly stained with Rhod-FF or Oregon Green Bapta-1 AM fluorescent dyes measuring mitochondrial and cytosolic [Ca 2+ ], respectively. False colour was applied to visualize the differences in the fluorescence intensities reflecting [Ca 2+ ] changes. Dark blue: low [Ca 2+ ]; yellow: high [Ca 2+ ]. Scale bar, 200 μm. ( b ) Histograms showing fold changes in the Rhod-FF/Oregon Green Bapta-1 AM fluorescence intensities of bclwav morphants compared with controlMO (mean±s.d. ; three independent experiments; * P <0.01, Student’s t -test). ( c ) Confocal stacks of controlMO versus bclwav MO embryos stained with Rhod-FF dye at 75% epiboly. The enveloping cell layer (EVL), deep cell layer (DCL) and YSL of the embryo were analysed. Fluorescence intensities were visualized with false colour. Scale bar, 50 μm. ( d ) Representative response of transfected HeLa cells loaded with the mitochondrial Ca 2+ -sensitive dye Rhod-2. Mitochondrial Ca 2+ uptake was stimulated with 5 μM thapsigargin (black arrow). Scale bar, 60 s. ( e ) Histograms depicting the quantitative response of the cells to 5 μM thapsigargin (mean±s.d. ; three independent experiments). ( f ) Analysis of the capacity of purified mitochondria from bclwav MO-, controlMO- or NADH (2 mM)-treated embryos (75% epiboly) to take up exogenous Ca 2+ (20 μM CaCl 2 ). Calcium Green 5N fluorescent dye was used to measure the decrease in extramitochondrial [Ca 2+ ], which directly reflects the mitochondrial uptake. Results are representative of two independent experiments. Scale bar, 60 s. ( g ) Histogram showing the capacity of purified mitochondria to uptake exogenous Ca 2+ as represented by a decrease in Oregon Green 5N fluorescence intensity (FI)/second. Results are representative of two independent experiments. ( h ) Bcl-wav co-immunoprecipitates with endogenous zVDAC1 in purified mitochondria from zebrafish embryos. Immunoprecipitations were performed using homogeneity-purified mitochondrial extracts from embryos (30% epiboly). Left lane (Mock), non-injected embryos; right lane (Flag-Bcl-wav), embryos injected with Flag-tagged bclwav transcripts. In both samples, two non-specific bands are revealed by the anti-VDAC1 antibody, the lower corresponding to the immunoglobulin light chain (black stars); however, in the sample prepared from embryos injected with Flag-tagged bclwav transcripts, a 34-kDa band corresponding to zVDAC1 can be detected (red arrow). ( i ) Bcl-wav interacts with endogenous VDAC1 via its BH4 domain in cellulo . Immunoprecipitation experiments were performed with protein extracts from transfected HeLa cells. Flag-Bcl-wav and Flag-Bcl-wavΔTM were both able to interact with VDAC1 (upper red arrow) but not Flag-ΔBH4Bcl-wav; the FlagBH4 peptide domain also interacted with VDAC1 (lower red arrow). ( j ) Histograms showing the percentage of embryos with the bent notochord phenotype (26 hpf) among bclwav morphants co-injected with ΔBH4bclwav mRNA or ΔBH4bclwav mRNA alone (mean±s.d. ; three independent experiments). ( k ) Histograms indicating the fold changes in Oregon Green Bapta-1 fluorescence intensity of bclwav morphants injected or not with ΔBH4Bclwav mRNA compared with controlMO (mean±s.d. ; three independent experiments; * P <0.01, Student’s t -test). Full scans of western blots can be found in Supplementary Fig. S10 . Full size image C&E movements strongly depend on mitochondrial Ca 2+ uptake Ca 2+ acts as a major intracellular messenger that controls different cellular processes and has a critical role during zebrafish development [12] . It has been clearly established that cytosolic Ca 2+ levels control actin dynamics and contribute to C&E movements in Xenopus and zebrafish [24] , [25] . Our results strongly suggest that the migration defects observed following bclwav silencing were due to a decrease in mitochondrial Ca 2+ uptake and subsequent Ca 2+ accumulation in the cytosol. To confirm this hypothesis, we directly tested whether disrupting mitochondrial Ca 2+ uptake would lead to the same C&E alterations as observed in bclwav MO. To this end, we knocked down the mcu , which was recently reported to be the major Ca 2+ carrier in the inner mitochondrial membrane [6] , [7] . Mcu silencing increased cytosolic Ca 2+ levels and decreased mitochondrial Ca 2+ levels ( Fig. 7a ), which correlated with major developmental alterations, including notochord deviation and anteroposterior axis reduction ( Fig. 7b,c ). Moreover, mcu knockdown also compromised blastomere migration ( Fig. 7d ) and altered F-actin dynamics and orientation ( Fig. 7f,g ), thus phenocopying the bclwav knockdown ( Supplementary Movie 5 ). It should be noted that the concurrent silencing of mcu and bclwav did not cause additive developmental defects ( Supplementary Fig. S6 ). 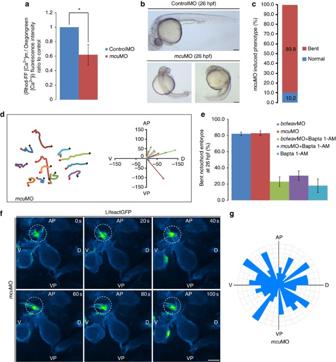Figure 7:Mcuknockdown phenocopiesbclwavsilencing. (a) Histograms indicating the fold changes in fluorescence intensity (Rhod-FF/Oregon Green Bapta-1 AM ratio) ofmcumorphants compared with controlMO embryos (mean±s.d.; three independent experiments; *P<0.01, Student’st-test). (b) Representative bright field images ofmcuMO at 26 hpf showing reduced anteroposterior axis formation and notochord deviation; these phenotypes are macroscopically identical to those observed inbclwavmorphants. Scale bar, 200 μm. (c) Histogram showing the percentage of abnormal phenotypes (bent notochord phenotype) resulting frommcuMO injection at 26 hpf. (d) Cell paths and vector projections of single mesodermal cells observed during C&E movements at the 75% epiboly stage in embryos injected withmcuMO, showing random cell migration. Vector projections are oriented as follows: AP, animal pole; D, dorsal; V, ventral; and VP, vegetal pole. (e) Histograms showing the percentage ofbclwavMO embryos (blue),mcuMO embryos (red),bclwavandmcumorphants injected with Bapta-1 AM (green and purple, respectively) or Bapta-1 AM alone (light blue) at 26 hpf with the bent notochord phenotype (mean±s.d.; three independent experiments). (f) Confocal spinning disk analysis of F-actin dynamics ofmcumorphants expressing lifeactgfpat the 75% epiboly stage, showing the location (white circles) and kinetics (seconds, bottom right corner) of F-actin polymerization. Image acquisition was performed on a single confocal section to visualize polymerized actin in lateral mesodermal cells. Scale bar, 10 μm. (g) Circular rose diagram ofmcuMO embryos representing the orientation of actin protrusions. This diagram shows the frequency of protrusions with a given orientation. InmcuMO embryos, the direction of F-actin protrusions is randomized compared with control embryo. Diagrams are oriented as follows: AP, animal pole; D, dorsal; V, ventral; and VP, vegetal pole. Figure 7: Mcu knockdown phenocopies bclwav silencing. ( a ) Histograms indicating the fold changes in fluorescence intensity (Rhod-FF/Oregon Green Bapta-1 AM ratio) of mcu morphants compared with controlMO embryos (mean±s.d. ; three independent experiments; * P <0.01, Student’s t -test). ( b ) Representative bright field images of mcu MO at 26 hpf showing reduced anteroposterior axis formation and notochord deviation; these phenotypes are macroscopically identical to those observed in bclwav morphants. Scale bar, 200 μm. ( c ) Histogram showing the percentage of abnormal phenotypes (bent notochord phenotype) resulting from mcu MO injection at 26 hpf. ( d ) Cell paths and vector projections of single mesodermal cells observed during C&E movements at the 75% epiboly stage in embryos injected with mcu MO, showing random cell migration. Vector projections are oriented as follows: AP, animal pole; D, dorsal; V, ventral; and VP, vegetal pole. ( e ) Histograms showing the percentage of bclwav MO embryos (blue), mcu MO embryos (red), bclwav and mcu morphants injected with Bapta-1 AM (green and purple, respectively) or Bapta-1 AM alone (light blue) at 26 hpf with the bent notochord phenotype (mean±s.d. ; three independent experiments). ( f ) Confocal spinning disk analysis of F-actin dynamics of mcu morphants expressing lifeact gfp at the 75% epiboly stage, showing the location (white circles) and kinetics (seconds, bottom right corner) of F-actin polymerization. Image acquisition was performed on a single confocal section to visualize polymerized actin in lateral mesodermal cells. Scale bar, 10 μm. ( g ) Circular rose diagram of mcu MO embryos representing the orientation of actin protrusions. This diagram shows the frequency of protrusions with a given orientation. In mcu MO embryos, the direction of F-actin protrusions is randomized compared with control embryo. Diagrams are oriented as follows: AP, animal pole; D, dorsal; V, ventral; and VP, vegetal pole. Full size image Conversely, we observed that the ‘bent notochord’ phenotype of the bclwav and mcu morphants could be rescued by co-injecting the EGTA derivative Bapta-1 AM, an efficient chelator of free Ca 2+ ( Fig. 7e ). These results suggest that the developmental abnormalities observed in morphant embryos were the direct consequence of Ca 2+ -trafficking alterations in blastomeres. During early zebrafish development, Ca 2+ signalling is primordial during morphogenetic movements [26] . Moreover, C&E movements appear to be partially under the control of the Wnt/PCP pathway and small GTPases such as RhoaA; thus, these movements could be regulated by calcium signalling [9] , [27] . We therefore investigated the effect of mcu knockdown on RhoA activation in human cells using a Rhotekin pull-down experiment. The efficiency of the small interfering RNA used in these experiments was previously validated in cellulo ( Supplementary Fig. S7 ). The level of active RhoA was significantly lower in mcu -silenced cells than in control cells ( Supplementary Fig. S8 ). Together, these results suggest that the cytosolic calcium accumulation observed in bclwav and mcu morphants may be responsible, at least in part, for the observed alteration of F-actin remodelling. Bcl-wav/VDAC1/MCU complex controls mitochondrial Ca 2+ uptake Finally, we performed a set of in cellulo experiments to better characterize the effect of Bcl-wav on mitochondrial Ca 2+ uptake. Bcl-wav was unable to increase mitochondrial Ca 2+ uptake ( Fig. 8a,b ) in an mcu- or/and vdac1 -null background, suggesting that VDAC1 and MCU may form a multiprotein Ca 2+ channel that controls Ca 2+ trafficking and blastomere movements during gastrulation. Indeed, Bcl-wav directly interacted with both VDAC1 and MCU, as shown by co-immunoprecipitation experiments in HeLa cells, suggesting that such interactions may also occur in the developing zebrafish ( Fig. 8c,d ). Importantly, contrary to the effects on mitochondrial Ca 2+ uptake, the pro-apoptotic effect of Bcl-wav seems to be MCU independent. Indeed, Bcl-wav can still activate caspase 3 and induce PARP cleavage in mcu knockdown cells ( Fig. 8e ) or in mcu morphant embryos ( Fig. 8f ), and ΔBH4Bcl-wav, which does not interact with VDAC1, was fully pro-apoptotic ( Supplementary Fig. S2c ). Consistent with these observations, a Bapta-1 AM probe was unable to rescue the embryonic mortality induced by bclwav mRNA ( Fig. 8g ). 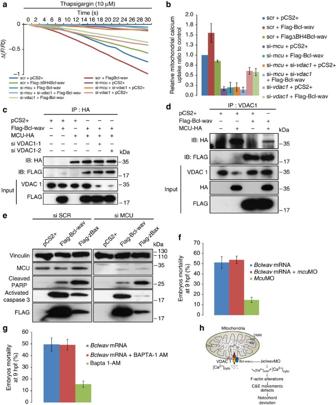Figure 8: The control of mitochondrial calcium by Bcl-wav, but not the induction of apoptosis, is VDAC1/MCU dependent. (a) Representative response of HeLa cells loaded with the intracellular Ca2+-sensitive dye FluoForte and stimulated with 10 μM thapsigargin. The ΔF/F0 decrease represents the mitochondrial calcium uptake measured during a 30-s period after the maximum of fluorescence intensity was reached. Cells were transfected with control scrambled (scr-),vdac1(si-vdac1),mcu(si-mcu)or si-vdac1+si-mcusmall interfering RNAs in combination with empty vector (pCS2+), pCS2+Flag-Bcl-wav or pCS2+Flag-ΔBH4Bcl-wav. (b) Mitochondrial calcium uptake induced by Bcl-wav is VDAC1/MCU dependent. Histogram plot representing the relative calcium uptake during 30 s after the maximum fluorescence intensity was achieved, normalized to that in scr+ pCS2+ cells (mean±s.d.; three independent experiments). (c) Bcl-wav interacts with MCU-HAin cellulo. Co-immunoprecipitation was performed in protein extracts from HeLa cells (scr, si1- or si2-vdac1) transfected with pCS2+Flag-Bcl-wav and pCS2+MCU-HA using anti-HA antibody. Effiency of si-vdac1was confirmed using an anti-VDAC1 antibody. (d) Bcl-wav, VDAC1 and MCU form a protein complex at the mitochondria. Immunoprecipitation of endogenous VDAC1 was performed in HeLa cells expressing the empty vector (pCS2+), Flag-Bcl-wav and/or MCU-HA. Both Flag-Bcl-wav and MCU-HA were detected in the co-transfected sample. (e) The pro-apoptotic activity of Bcl-wav is MCU independent. Caspase 3 is activated, and PARP is cleaved in both scr- and si-mcuHeLa cells transfected with pCS2+Flag-Bcl-wav and pCS2+Flag-ΔBH4Bcl-wav; this result is not observed in control cells. Vinculin protein was used for calibration purposes. HeLa cells transfected with pCS2+Flag-zBax were used as positive controls. (f) Overexpression ofbclwavis lethal inmcumorphant embryos. The injection ofbclwavmRNA into WT ormcuMO embryos at the one-cell stage induces early mortality during gastrulation (mean±s.d.; three independent experiments). (g) Histograms showing the percentage mortality of embryos injected withbclwavmRNA and Bapta-1 AM, alone or in combination (mean±s.d.; three independent experiments), at 9 hpf. (h) Model of Bcl-wav function during early zebrafish development. At mitochondria, Bcl-wav interacts with zVDAC1 and MCU to control Ca2+entry.Bclwavknockdown increases free cytosolic Ca2+levels, which may alter actin cytoskeletal dynamics, leading to changes in C&E movements and subsequent notochord deviation. Full scans of western blots are provided inSupplementary Fig. S11. Figure 8: The control of mitochondrial calcium by Bcl-wav, but not the induction of apoptosis, is VDAC1/MCU dependent. ( a ) Representative response of HeLa cells loaded with the intracellular Ca 2+ -sensitive dye FluoForte and stimulated with 10 μM thapsigargin. The ΔF/F0 decrease represents the mitochondrial calcium uptake measured during a 30-s period after the maximum of fluorescence intensity was reached. Cells were transfected with control scrambled (scr-), vdac1 (si- vdac1) , mcu (si- mcu) or si- vdac1 +si- mcu small interfering RNAs in combination with empty vector (pCS2+), pCS2+Flag-Bcl-wav or pCS2+Flag-ΔBH4Bcl-wav. ( b ) Mitochondrial calcium uptake induced by Bcl-wav is VDAC1/MCU dependent. Histogram plot representing the relative calcium uptake during 30 s after the maximum fluorescence intensity was achieved, normalized to that in scr+ pCS2+ cells (mean±s.d. ; three independent experiments). ( c ) Bcl-wav interacts with MCU-HA in cellulo . Co-immunoprecipitation was performed in protein extracts from HeLa cells (scr, si1- or si2- vdac1 ) transfected with pCS2+Flag-Bcl-wav and pCS2+MCU-HA using anti-HA antibody. Effiency of si- vdac1 was confirmed using an anti-VDAC1 antibody. ( d ) Bcl-wav, VDAC1 and MCU form a protein complex at the mitochondria. Immunoprecipitation of endogenous VDAC1 was performed in HeLa cells expressing the empty vector (pCS2+), Flag-Bcl-wav and/or MCU-HA. Both Flag-Bcl-wav and MCU-HA were detected in the co-transfected sample. ( e ) The pro-apoptotic activity of Bcl-wav is MCU independent. Caspase 3 is activated, and PARP is cleaved in both scr- and si- mcu HeLa cells transfected with pCS2+Flag-Bcl-wav and pCS2+Flag-ΔBH4Bcl-wav; this result is not observed in control cells. Vinculin protein was used for calibration purposes. HeLa cells transfected with pCS2+Flag-zBax were used as positive controls. ( f ) Overexpression of bclwav is lethal in mcu morphant embryos. The injection of bclwav mRNA into WT or mcu MO embryos at the one-cell stage induces early mortality during gastrulation (mean±s.d. ; three independent experiments). ( g ) Histograms showing the percentage mortality of embryos injected with bclwav mRNA and Bapta-1 AM, alone or in combination (mean±s.d. ; three independent experiments), at 9 hpf. ( h ) Model of Bcl-wav function during early zebrafish development. At mitochondria, Bcl-wav interacts with zVDAC1 and MCU to control Ca 2+ entry. Bclwav knockdown increases free cytosolic Ca 2+ levels, which may alter actin cytoskeletal dynamics, leading to changes in C&E movements and subsequent notochord deviation. Full scans of western blots are provided in Supplementary Fig. S11 . Full size image Taken together, these results show that Bcl-wav enhances Ca 2+ uptake into the mitochondria via VDAC1 and MCU and may accelerate apoptosis by activating Bax. During gastrulation, Bcl-wav and MCU serve as key factors in C&E movements by controlling mitochondrial Ca 2+ trafficking and the dynamics of F-actin protrusions in migrating blastomeres ( Fig. 8h ). Here we report the identification and functional characterization of Bcl-wav, a new member of the multidomain Bcl-2 family of apoptosis regulators. This gene was identified using profile-based hidden Markov models, combining sequence and three-dimensional structure information [15] . Interestingly, Bcl-wav was found in aquatic egg-laying species (teleosts and anurans) but not in mammals or birds, suggesting that Bcl-wav was evolutionarily selected for a specific role in the particular reproductive process of these egg-laying species. Indeed, some Bcl-2 members seem to have specialized roles in the control of oocyte survival and early embryo development [13] , [28] , [29] , [30] . Combined bioinformatic and functional analyses identified Bcl-wav as a new multidomain Bcl-2 member [31] . We showed that Bcl-wav is able to bind to Bax and subsequently induce caspase activation. Thus, Bcl-wav seems to be an atypical member of the subfamily of multidomain death accelerators. The Bcl-wav protein is mostly a mitochondrial resident, suggesting that it may share some functional similarities with Bak, a multidomain protein that is not expressed during zebrafish development [11] . In this regard, Bcl-wav is able to interact with VDAC1, a property shared with Bak [9] , [32] . VDAC1 is known to permit Ca 2+ transfer from the cytosol to the mitochondrial matrix [19] . This suggests that Bcl-wav could have a role in the control of intracellular Ca 2+ fluxes. Bclwav knockdown resulted in a marked decrease in mitochondrial Ca 2+ levels, together with an increase in cytosolic Ca 2+ . Interestingly, knockdown of mcu also induced marked increases in cytosolic Ca 2+ and phenocopied the bclwav knockdown phenotype, which not only demonstrates the critical role of MCU in vertebrate development but also suggests the existence of a multiprotein Ca 2+ channel composed of VDAC1 and MCU. Indeed, Bcl-wav can interact with both VDAC1 and MCU, and these proteins can also interact with each other. In addition, the effect of Bcl-wav on mitochondrial calcium uptake depends on both VDAC1 and MCU. Thus, at the molecular level, it may be speculated that Bcl-wav maintains the VDAC1/MCU channel in an ‘open state’, allowing Ca 2+ entry into the mitochondrial matrix. In this way, the fine-tuning of mitochondrial Ca 2+ fluxes might be ensured by the combined effects of apoptosis accelerators, including Bcl-wav, and apoptosis inhibitors, such as Bcl-xL, on the permeability of the VDAC1 Ca 2+ channel. In fact, Bax itself was reported to interact with VDAC [33] , but also Bcl-xL [21] that can modulate its permeability [22] . Our data support the model that Bcl-xL is able to inhibit massive Ca 2+ entry into mitochondria. In this respect, it would be interesting to evaluate the existence of a ‘ménage à trois’ between Bcl-wav, Bcl-xL and VDAC1. The observed phenotypes of bclwav and mcu morphants may tentatively be attributed, at least in part, to the observed effects on cytosolic and mitochondrial Ca 2+ pools. Indeed, during zebrafish gastrulation, C&E movements appear to be partially under the control of the Wnt/PCP pathway [34] , [35] . This pathway activates small GTPases such as RhoA and Rac1, which are responsible for F-actin dynamics and polarization [36] . Given that RhoA activation is decreased in mcu null cells, we hypothesize that bclwav and mcu silencing in zebrafish impair F-actin dynamics by altering Rho GTPase activity. Indeed, it has been demonstrated that an increase in cytosolic Ca 2+ modulates Rac1 and RhoA activities, leading to alterations in cell migration and reversing the orientation of protrusions in neuronal cells [36] . Interestingly, components of the Wnt/PCP pathway can also modulate Ca 2+ signalling [37] , [38] . These data are consistent with observations in zebrafish, showing that throughout gastrulation Ca 2+ waves occur in the vicinity of the dorsal axis of the embryo, where C&E movements take place [39] . During these Ca 2+ waves, cells are exposed to high Ca 2+ concentrations, which may be detrimental; thus, mitochondrial Ca 2+ uptake is presumably critical for maintaining Ca 2+ homoeostasis in migrating blastomeres. In bclwav and mcu morphants, mitochondrial Ca 2+ uptake appears to be compromised, as suggested by decreased mitochondrial Ca 2+ levels; this may in turn explain the observed cytosolic Ca 2+ increase. Thus, bclwav knockdown may alter C&E movements via its effects on temporal and spatial Ca 2+ signalling in the gastrula. This hypothesis accounts for the observed disruption of the distribution of ntl -positive cells in these morphants and the subsequent malformations. It was recently shown that embryos that are deficient in components of the Wnt/PCP pathway and thus have abnormal C&E movements also exhibited defects in somite and notochord formation [40] . Together, our results support the hypothesis that Bcl-wav orchestrates morphogenetic movements by acting on intracellular Ca 2+ trafficking via its interactions with VDAC1/MCU. These data raise the possibility that the primary role of Bcl-2 proteins during development might be to maintain cytoskeletal dynamics by regulating intracellular Ca 2+ fluxes. From an evolutionary point of view, the Bcl-2 family might be linked to the appearance of gastrulation in metazoans. Zebrafish care Experimental procedures followed the recommendations of the French Council on Animal Care (Arrêté du 27 décembre 1994). Protocols were approved by the Committee for animal experimentation Université Claude Bernard Lyon 1. Zebrafish (AB/TU and AB/TL strains) were raised and maintained at 28.5 °C according to the standard procedures. Embryos were collected after fertilization and injected at the one-cell stage. Morpholinos and mRNA Morpholinos were designed according to the manufacturer’s recommendations (Gene Tools, Philomath, OR, USA): bclwav MO1 (5′-CATCAGCTCAGATACACACAGGTCA-3′) hybridizes with bclwav mRNA from position −22 to +3 relative to the start codon; bclwav MO2 (5′-TCACAGCGTCGTCTGACCGTCCCAT-3′) hybridizes with bclwav mRNA from position +1 to position +25. We used the bclwav MO1 with five mismatches (underlined) as negative control: 5mis-MO (5′-C G TCAG A TC G GATAC T CACAGGT T A-3′). Other morpholinos included p53 -MO (5′-GCGCCATTGCTTTGCAAGAATTG-3′), mcu MO (5′-CATCTCTGAAGTGAAACCCGGCCGA-3′) and mcu -5mis-MO (5′-GAGCTATGAATTGAAACTCGGACGA-3′). Details regarding bclwav cloning (primer sequences are listed in Supplementary Table S1 ) and small interfering RNA experiments are provided in Supplementary Methods . Bcl-wav protein and antibody production The Bcl-wav protein (residues 1–177) was produced in BL-21 (DE3) bacteria, purified on a Ni-NTA-agarose column [41] and subsequently used for polyclonal antibody production (Valbex, Villeurbanne). Rabbit serum immunoglobulin was purified on a protein A-agarose affinity column [42] . In situ hybridization For bclwav expression analysis, three probes were used: two were partial and non-overlapping ( bclwav 1–293 from position +1 to +293 and bclwav 300–600 from position +300 to +600), and one represented full-length bclwav. Briefly, digoxigenin-labelled riboprobes were synthesized from pCS2+ bclwav , pCS2+ bclwav 1–293 , pCS2+ bclwav 300–600 , pCS2+ ntl and pCS2+ col2.1a . After permeabilization, embryos were hybridized overnight. Then, embryos were incubated with an anti-digoxigenin antibody (Roche; 1:10,000), stained and observed under a Leica MZ6 stereo-microscope [43] . Subcellular fractionation All steps were carried out at 4 °C. Blastomere mitochondria, mitochondria and ER localized to the YSL of different embryo stages (before mid-blastula transition, sphere, 30%, 50% and 75% epiboly progression) were purified as follows: 100 embryos were added to 1 ml of cold MB buffer (210 mM mannitol, 70 mM sucrose, 1 mM EDTA and 10 mM HEPES (pH 7.5) containing protease inhibitors), and the yolk sac was disrupted by pipetting up and down. Embryos were centrifuged for 2 min at 300 g to separate blastomeres and yolk cells. The pellet, containing blastomeres, was resuspended in 1 ml of MB buffer, and the cells were disrupted by shearing with a 1-ml syringe and a 26 G × 2/3 needle 50 times. The disrupted blastomeres and yolk cells were then centrifuged twice at 1,500 g for 5 min to eliminate nuclei and finally centrifuged at 10,600 g to pellet the mitochondria. Mitochondria were washed with 1 ml of MB buffer and resuspended in an appropriate volume of MB buffer for further analyses. The supernatant was centrifuged at 100,000 × g for 1 h, and the pellet containing the ER fraction was resuspended in RIPA buffer for further analysis. Cell death assays To study Bcl-wav pro-apoptotic activity, HeLa cells were transiently transfected with appropriate constructs and treated with dimethyl sulphoxide (DMSO) or 10 μM thapsigargin 24 h later. Then, 24 h after drug treatment, cell death was quantified by annexin-V-Cy3 (Biovision) staining according to the manufacturer’s protocols followed by flow-cytometry analysis using a FACScan (Becton Dickinson). Data were processed using CellQuest Pro software. To analyse the effect of Bcl-wav on caspase activation, HeLa cells were transiently transfected with appropriate constructs alone or in combination. Twenty-four hours later, caspase-positive cells were labelled using the FLICA detection kit (ImmunoChemistry Technologies LLC). Pycnotic nuclei were labelled using Hoechst 33342. Cells were observed under a fluorescent microscope, and the percentages of caspase-positive and Hoechst-positive cells were determined (~100 cells per field). For terminal deoxynucleotidyl transferase-mediated dUTP nick end-labelling assays, embryos were fixed in 4% paraformaldehyde in PBS overnight at 4 °C, washed at room temperature and stored in methanol at −20 °C. After progressive rehydratation in PBS, embryos were washed four times in PBS, 0.1% Tween 20 (5 min per wash). Permeabilization was performed for 15 min in PBS, 0.1% Triton X-100 and 0.1% sodium citrate at +4 °C, cell death was quantitated using the POD in situ cell death detection kit (Roche). Cell death was detected by measuring the incorporation of FITC-labelled nucleotides by confocal microscopy. For zebrafish caspase 3 assay, embryos (50% epiboly) were fixed in 4% paraformaldehyde overnight at 4 °C and stored in 100% methanol at −20 °C. After progressive rehydratation in PBS, embryos were washed three times for 10 min in PBS+0.1% Tween (PBST) and subsequently soaked for 1 h in blocking solution (10% heat-inactivated FBS and 3% BSA in PBST). Embryos were then incubated overnight at +4 °C with anti-activated caspase 3 antibody (1/500). Following three washes in PBST, 0.3% Triton and 1% DMSO, embryos were soaked in blocking solution for 1 h. Embryos were then incubated overnight at +4 °C with a goat anti-rabbit red fluorescent antibody (1/200 in blocking solution). Embryos were washed three times in 0.3% Triton X-100 and 1% DMSO in PBST, incubated with Hoechst 33342 (1/10,000) for 30 min, washed with 1 × PBS and stored in 80% glycerol. Embryos were analysed using a Nikon TE300 fluorescence microscope. Immunoprecipitation For zebrafish embryo immunoprecipitation experiments, mitochondria from embryos injected with or without Flag-Bcl-wav mRNA at 30% epiboly were purified as described above. Mitochondria were resuspended in 1% CHAPS buffer (1% CHAPS, 150 mM NaCl, 50 mM Tris (pH 7.4) and protease inhibitors). Extracts were precleared with protein G-Sepharose beads for 2 h at 4 °C, and then 100 μg of mitochondria was incubated with 5 μg of anti-Flag M2 overnight. Extracts were then incubated for 3 h with 15 μl of protein G-Sepharose beads and centrifuged for 5 min at 5,000 r.p.m. Collected beads containing immunoprecipitated fractions were washed three times in CHAPS buffer, resuspended in SDS–PAGE sample buffer and analysed by immunoblotting using anti-VDAC1 antibody. For HeLa cell immunoprecipitation experiments, 8 × 10 6 HeLa cells were transfected with the appropriate constructs. After 24 h, cells were lysed in TNE buffer (10 mM Tris-HCl, 200 mM NaCl, 1 mM EDTA (pH 7.4), 1 mM β-glycerophosphate, 1 mM orthovanadate, 0.1 mM sodium pyrophosphate and protease inhibitors). Extracts were precleared with protein G-Sepharose beads and subsequently incubated overnight with 3 μg of anti-VDAC1 or 1 μg of anti-HA antibodies. Extracts were then incubated for 3 h with protein G-Sepharose beads and centrifuged for 5 min at 5,000 r.p.m. Pellets containing immunoprecipitated fractions were washed five times in TNE buffer and analysed by immunoblotting. The RhoA activation assay is described in Supplementary Methods . In vivo staining For cytosolic and mitochondrial Ca 2+ measurements, one-cell stage embryos were injected with 10 μM Oregon Green 488 Bapta-1 AM or 10 μM Rhod-FF, alone or in combination with RNA or morpholinos. Embryos were then analysed at 75% epiboly using a Nikon TE300 fluorescence microscope. For mitochondrial Ca 2+ measurements in the YSL, enveloping layer and deep cell layer, one-cell stage was injected with 250 μM Rhod-FF with controlMO or bclwav MO. Embryos were incubated at 28.5 °C and subsequently analysed at 50–75% epiboly using a Zeiss 780 confocal microscope to specifically visualize each cell population. Images were acquired from 49 stacks of 4 μm each per embryo. For F-actin staining, embryos were fixed overnight in 4% paraformaldehyde at 4 °C and incubated with phalloidin [44] . Active mitochondria at the 50% epiboly stage were stained by incubating embryos for 30 min in 500 nM Mitotracker Red at 28.5 °C. Embryos were washed three times and visualized using a Nikon TE300 microscope. Image acquisition was carried out with the same gain, amplification and exposure time for each experimental condition and corresponding control. Images were analysed using ImageJ software. Mitochondrial calcium measurements in HeLa cells Mitochondrial calcium in HeLa cells, transiently transfected with pCS2+, pCS2+Flag-Bcl-wav and pCS2+Flag-zBcl-xL, was measured by monitoring Rhod-2 fluorescence in cells cultured in 96-well plates using a Mithras LB 940 multimode microplate reader (Berthold Technologies). Cells were loaded with 5 μM Rhod-2 acetoxymethyl ester (Molecular Probes) in balanced salt solution (BBS) (121 mM NaCl, 5.4 mM KCl, 0.8 mM MgCl 2 , 1.8 mM CaCl 2 , 6 mM NaHCO 3 , 5.5 mM D-glucose and 25 mM HEPES, pH 7.3) for 45 min at 37 °C. Following Rhod-2 loading, cells were incubated a further 30 min in fresh Ca 2+ -free BBS at room temperature for dye de-esterification. Fluorescence values were obtained by excitation at 550 nm, and emission signal was collected at 580 nm every 400 ms. Thapsigargin in Ca 2+ -free BBS was injected in each well after 15 s of measurement at a final concentration of 5 μM. Extramitochondrial free Ca 2+ was monitored in scr-, si- mcu and/or si- vdac1 HeLa cells transiently transfected with pCS2+, Flag-Bcl-wav or Flag-ΔBH4Bcl-wav using the FluoForte probe (Enzo). Cells were loaded with 5 μM FluoForte for 1 h at 37 °C in fresh Ca 2+ -free BBS. Fluoforte fluorescence was monitored every 2 s using a Zeiss 780 confocal microscope after thapsigargin injection (10 μM final). Relative mitochondrial calcium uptake was calculated by computing linear fits for 30 s after the maximum fluorescence intensity was reached. Calcium uptake capacity of isolated zebrafish mitochondria Extramitochondrial free Ca 2+ was monitored in the presence of isolated mitochondria using Oregon Green 5N hexapotassium salt. Purified mitochondria from 75% epiboly embryos were resuspended in KCl medium (125 mM KCl, 2 mM K 2 HPO 4 , 1 mM MgCl 2 and 20 mM HEPES, pH 7) containing 1 μM Oregon Green 5N (Molecular Probes) and supplemented with 5 mM glutamate and 5 mM malate. Oregon Green 5N fluorescence was measured using a Mithras LB 940 multimode microplate reader (Berthold Technologies) with excitation at 485 nm and emission at 510 nm. CaCl 2 (in supplemented KCl medium) was injected after 30 s of measurement at a final concentration of 20 μM. Time-lapse microscopy For cell tracing experiments, embryos co-injected with controlMO or bclwav MO and lifeactgfp mRNA were manually dechorionated at the shield stage and incorporated into 0.5% low-melting point agarose. Before solidification, embryos were orientated in the dorsoventral plane to permit observation of the lateral mesoderm. Embryos were then observed using a Leica DMI4000 inverted microscope equipped with a 28°C observation chamber, an EMCCD camera (Photometrics Quantem 512) and a × 40 oil immersion objective. Time-lapse images were acquired every 20 s, and total acquisition time was 20 min. Image analyses were performed using ImageJ. Transplantation Embryos expressing β-actin-GFP were used as control donors, whereas bclwav MO was co-injected with rhodamine. Cells from control and morphant donors were removed at 50% epiboly and transplanted into the shield of the same WT receiver embryo at shield stage. Transplantation was verified under a fluorescence microscope. Cell migration in receiver embryos was analysed at 90% epiboly. Statistical analyses Error bars displayed on graphs represent the means±s.d. of three independent experiments. Statistical significance was analysed using Student’s t -test. P <0.01 was considered significant. Co-localization percentage Co-localization percentage between Flag-Bcl-wav and mitochondria labelled with MitoTracker was calculated with Zen software. Details regarding subcellular localization experiments are provided in Supplementary Methods . Accession codes: Sequence data have been deposited in GenBank/EMBL/DDBJ under accession number GU350411.1 . How to cite this article: Prudent, J. et al . Bcl-wav and the mitochondrial calcium uniporter drive gastrula morphogenesis in zebrafish. Nat. Commun. 4:2330 doi: 10.1038/ncomms3330 (2013).